Tracking the origin of two genetic components associated with transposable element bursts in domesticated rice Transposable elements (TEs) shape genome evolution through periodic bursts of amplification. In this study prior knowledge of the mPing/Ping/Pong TE family is exploited to track their copy numbers and distribution in genome sequences from 3,000 accessions of domesticated Oryza sativa (rice) and the wild progenitor Oryza rufipogon . We find that mPing bursts are restricted to recent domestication and is likely due to the accumulation of two TE components, Ping16A and Ping16A_Stow , that appear to be critical for mPing hyperactivity. Ping16A is a variant of the autonomous element with reduced activity as shown in a yeast transposition assay. Transposition of Ping16A into a Stowaway element generated Ping16A_Stow , the only Ping locus shared by all bursting accessions, and shown here to correlate with high mPing copies. Finally, we show that sustained activity of the mPing/Ping family in domesticated rice produced the components necessary for mPing bursts, not the loss of epigenetic regulation. Eukaryotic genomes are populated with transposable elements (TEs), many attaining copy numbers of hundreds to thousands of elements by rapid amplification, called a TE burst [1] . For a TE to successfully burst, it must be able to increase its copy number without killing its host or being silenced by host surveillance [2] , [3] . However, because the vast majority of TE bursts have been inferred after the fact—via computational analysis of whole-genome sequence—the stealth features they require for success have remained largely undiscovered [2] , [4] . Revealing these features requires the identification of a TE in the midst of a burst. This was accomplished for the miniature inverted-repeat TE (MITE) mPing from rice [5] , [6] . MITEs are nonautonomous DNA transposons that are the most common TE associated with the noncoding regions of plant genes [1] . To understand how MITEs attain high copy numbers, a computational approach was used to identify mPing , and its source of transposase, encoded by the related autonomous Ping element (Fig. 1a ) [5] . Fig. 1 Abundance of mPing , Ping , and Pong elements in rice and O. rufipogon . a Comparison of structures of mPing , Ping, and Pong . TIRs are indicated by black triangles. Two protein-coding genes ORF1 and ORF2 ( TPase ) encoded by Ping or Pong are indicated by dark gray boxes. Homologous regions between elements are connected by lines and percent identities are shown. The black star on Ping indicates the + 16 G/A SNP that differs between mPing and Ping16A . Copy numbers across the 3000 rice accessions of mPing ( b ), Ping ( c ), and Pong ( d ). The bar plot in the dashed box in b shows accessions with >50 mPing elements. e , mPing copy number of 48 O. rufipogon accessions. f Ping copy number of 48 O. rufipogon accessions. g Pong copy number of 48 O. rufipogon accessions. Source data for Fig. 1 b–g are provided in Supplementary Data 1 - 2 Full size image Ongoing bursts of mPing were discovered in four temperate japonica accessions: EG4, HEG4, A119, and A123, whose genomes were sequenced, and insertion sites and epigenetic landscape determined [6] , [7] , [8] . These analyses uncovered two features of successful mPing bursts. First, although mPing , like other DNA TEs, prefers genic insertions, de novo insertions in exons were only 14% of expected for random insertions, thus minimizing harm to the host [6] , [8] . Exon avoidance arises from mPing ’s extended 9-bp adenine-thymine (AT)-rich insertion preference [6] , [8] coupled with rice exon sequences that are significantly more guanine-cytosine (GC) rich than rice introns (51% vs. 37%) [9] . Second, because mPing does not share coding sequences with Ping (Fig. 1a ), increases in its copy number and host recognition of its sequences does not silence Ping genes, thus allowing the continuous production of the proteins necessary to sustain the burst for decades [7] . The contributions of two other genetic components to the success of the bursts could not be assessed previously and are a focus of this study. First, all Ping elements in the four bursting accessions contain a single nucleotide polymorphism (SNP) at position 16 ( + 16 G/A) that distinguishes mPing and Ping sequences (Fig. 1a ). The second genetic component is a single Ping locus (called Ping16A_Stow ) that is the only Ping locus shared by all bursting accessions [7] . Comparative sequence analysis of two of the four bursting accessions (A123 and A119) revealed that they were derived by self or sibling pollination about a century ago from a common ancestor that had not yet undergone Ping or mPing amplification [7] . Significantly, this common ancestor had only a single Ping locus, which was Ping16A_Stow [7] . To understand the origin of these genetic components and their possible role in the burst, we analyzed the presence, sequence, and copy numbers of Ping and mPing elements in the genomes of 3000 domesticated rice accessions and 48 genomes of their wild progenitor, Oryza rufipogon . Rice has been divided into five major subgroups ( indica , aus / boro , aromatic , temperate japonica , and tropical japonica ) that are thought to have originated from distinct populations of the wild progenitor O. rufipogon that arose prior to domestication [10] , [11] . Rice genomes are very stable: all analyzed genomes are composed of 12 chromosomes [12] , [13] , and rice subgroups share high sequence identity ( > 98.9%) [13] . However, the genomes also exhibit extensive presence–absence variation both within (5%) and between (10%–19%) subgroups [13] , [14] , with TEs representing more than half of this variation. In addition, significant gene flow from japonica to indica and aus has been noted previously, reflecting the more ancient origin of japonica [10] , [15] . Knowledge of the relationships between the major subgroups of rice and the populations of O. rufipogon have been utilized in this study to better understand the identity and origin of the components necessary for mPing bursts. Of particular interest was whether (i) mPing bursts could be detected in other accessions of wild and/or domesticated rice, (ii) the + 16 G/A Ping SNP and Ping16A_Stow could be detected in wild rice or first appeared in domesticated rice, and (iii) the presence of + 16 G/A Ping SNP and Ping16A_Stow correlated with higher mPing copy numbers. Finally, another potential player that may be implicated in mPing bursts, Pong , a related transposase-encoding element, is a focus of this study (Fig. 1a ). The Pong element is the closest relative of Ping and there are at least five identical copies found in the genome of all rice accessions analyzed to date [7] , [16] . Pong encoded proteins catalyzed the transposition of mPing in rice cell culture [5] and in transposition assays in Arabidopsis thaliana and yeast [17] , [18] . However, Pong elements do not catalyze mPing transposition in planta because all Pong copies are effectively silenced and its sequences are associated with heterochromatin [7] . Here we are able to address questions regarding the origin and stability of Pong silencing before and after domestication. Our analysis show that mPing copy number has burst only in a few domesticated accessions and is associated with the acquisition of two variants of the transposase loci, Ping16A and Ping16A_Stow . The proportion of accessions with Ping16A has increased in domesticated rice while the original Ping ( Ping16G ) has been dramatically reduced. A transposition event of Ping16A into a Stowaway element created Ping16A_Stow whose presence correlates with accessions that have high mPing copies. We reject the hypothesis that a loss of global epigenetic regulation has occurred as no other TEs have amplified, indicating that these new Ping loci are the primary driver of the observed mPing burst in domesticated rice. Detection of mPing, Ping , and Pong element Insertion sites and copy numbers for mPing , Ping , and Pong were identified from genome sequences of 3000 rice accessions using RelocaTE2 [19] (see Methods). The paired-end DNA libraries had an average insert size of ~ 500 bp and were sequenced to a depth of 14-fold genome coverage [20] , which allowed clear distinction between mPing, Ping, and Pong elements (Fig. 1a ). Sequence analyses identified a total of 27,535 mPings , 262 Pings , and 12,748 Pong s (Figs. 1 b–d and Supplementary Data 1 ). Copy numbers of mPing , Ping , and Pong elements in each genome were also estimated using a read depth method (see Methods). 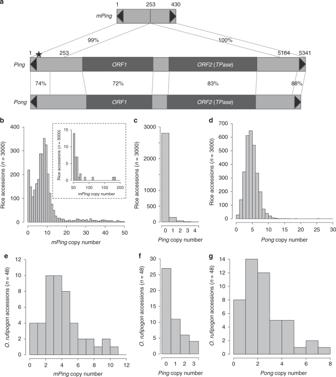Fig. 1 Abundance ofmPing,Ping, andPongelements in rice andO. rufipogon.aComparison of structures ofmPing,Ping,andPong. TIRs are indicated by black triangles. Two protein-coding genesORF1andORF2(TPase) encoded byPingorPongare indicated by dark gray boxes. Homologous regions between elements are connected by lines and percent identities are shown. The black star onPingindicates the + 16 G/A SNP that differs betweenmPingandPing16A. Copy numbers across the 3000 rice accessions ofmPing(b),Ping(c), andPong(d). The bar plot in the dashed box inbshows accessions with >50mPingelements.e,mPingcopy number of 48O. rufipogonaccessions.fPingcopy number of 48O. rufipogonaccessions.gPongcopy number of 48O. rufipogonaccessions.Source datafor Fig.1b–g are provided in Supplementary Data1-2 Outputs from the RelocaTE2 and read depth methods were well correlated (Pearson’s correlation, R = 0.97, P < 2.2e–16 for mPing ; R = 0.82, P < 2.2e–16 for Ping ; R = 0.66, P < 2.2e–16 for Pong ; Supplementary Figure 1 ) indicating that both methods to estimate approximate mPing , Ping , and Pong copy numbers in the 3000 rice accessions were robust. Insertion sites and copy numbers for mPing , Ping , and Pong were also identified for 48 O. rufipogon accessions, but only the read depth method was used because of the limited insert size of the libraries (Supplementary Data 2 ). In total, 195 mPing s , 25 Pings , and 125 Pongs were estimated to be present in the 48 O. rufipogon accessions (Supplementary Data 2 , Figs. 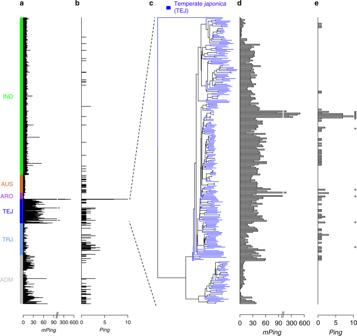Fig. 2 Copy numbers ofmPing, Ping, andPongelements in rice subgroups.amPingcopy numbers in 3000 genomes and the four accessions undergoingmPingbursts (HEG4, EG4, A119, and A123). Colors represent the five major rice subgroups:indica(IND),aus/boro(AUS),aromatic(ARO), temperatejaponica(TEJ), tropicaljaponica(TRJ), and admixed (ADM).bPingcopy numbers in 3000 genomes and the four accessions undergoingmPingbursts.cNeighbor-joining tree of temperatejaponicaaccessions using genome-wide SNPs.dmPingcopy number of temperatejaponicaaccessions.ePingcopy number of temperatejaponicaaccessions. Accessions that have thePing16A_Stowlocus are noted with open circles.Source datafor Fig.2a, b, d, eare provided in Supplementary Data1 1 e–g, and Supplementary Figure 2 ). Copy number variation of mPing and Ping elements None of the 3000 rice accessions analyzed in this study have more mPing elements than the 231–503 copies found in the four temperate japonica accessions (HEG4, EG4, A119, A123) in the midst of mPing bursts [7] . Of the 3000 rice accessions, 2780 (92.7%) contain mPing , with an average of about 9 elements per accession (Fig. 1b ). 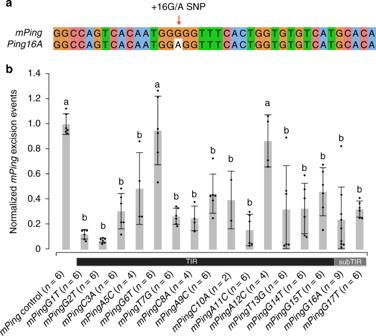Fig. 3 Transposition frequency ofmPingvariants in the yeast assay.aSequence alignment ofmPingandPing16Aterminal sequence (1–40 bp). The SNP betweenmPingandPing16Aat position 16 ( + 16 G/A SNP) is indicated by the red arrow.bTransposition frequency ofmPingvariants with mutations at the 5ʹ end in the yeast assay.Xaxis indicatesmPingvariants with mutations at 14 positions in the 5ʹ TIR and two positions outside the TIR. For example,mPingG16Arepresents anmPingvariant having a G-to-A mutation at position 16. A variantmPingC4Awas not included because the lack of qualified experiments.Yaxis shows transposition frequency that was measured asmPingexcision events per million cells and normalized to the controlmPing. The error bars show standard deviation (s.d.) of 2-9 independent biological replicates. Letters (a and b) above the bars indicate significant differences of transposition frequency betweenmPingvariants and control (adjustedP-value ≤ 0.05). The adjustedP-values are based on a one-way ANOVA (P-value = 2.37e–15,F-value = 12.34, DF = 16) followed by a Tukey’s honest significant difference (Tukey’s HSD) test.Source datafor Fig.3bare provided as aSource Datafile Temperate japonica accessions do, however, have significantly more mPing elements (~30.5/accession) than tropical japonica (~2.6/accession), indica (~8.2/accession), or aus/boro (~3.8/accession) (one-way analysis of variance (ANOVA) with Tukey’s honest significant difference (HSD) test, adjusted P -value < 2e–16; Supplementary Table 1 and Supplementary Figure 3 ). All O. rufipogon accessions have mPing elements with copy numbers ranging from 1 to 11 (mean = 4.06, standard deviation = 2.39; Fig. 1e and Supplementary Figure 2 ). 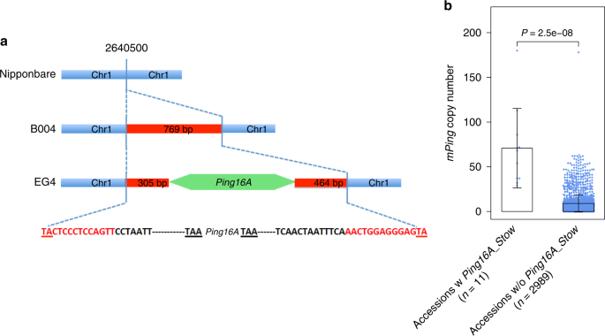Fig. 4 Structure of thePing16A_Stowlocus, which is associated with increasedmPingcopy number.aStructure of thePing16A_Stowinsertion site. ThePing16Aelement (green arrow) is inserted in the middle of a nonautonomousStowawayelement (red box), which is not in Nipponbare (blue bar). Nucleotides shown within the blue dotted lines are the sequences of the nonautonomousStowawayelement. Target site duplications (TSDs) are indicated by nucleotides underscored.bComparisons ofmPingcopy number in 3000 rice accessions with or withoutPing16A_Stowin the genome. Gray dots indicatemPingcopy number of rice accessions in each category. The error bars show standard deviation (s.d.) of each category. Differences inmPingcopy numbers between two categories were tested by a two-tailed Wilcoxon–Mann–Whitney test.Source datafor Fig.4bare provided in Supplementary Data1 Prior studies identified four subtypes of mPing elements ( mPingA-D ) in domesticated rice (Supplementary Figure 4 ) [5] , representing four distinct deletion derivatives of Ping . Two of the four subtypes ( mPingA , B ) were previously detected in O. rufipogon accessions [21] , [22] . Here we detected all four subtypes of mPing elements in O. rufipogon accessions (Supplementary Table 2 ) indicating that mPingA-D arose in O. rufipogon prior to domestication. Like mPing , none of the 3000 genomes analyzed in this study have more Ping elements (7–10) than the four accessions undergoing mPing bursts [7] . Ping elements were detected in only 199 of 3000 accessions (6.6%) (Fig. 2 and Table 1 ) with most of the 199 (74.8%) having only a single copy and two accessions having 4 Pings (Fig. 2b ). In contrast, Ping elements were detected in 21 of 48 (43.7%) of the O. rufipogon accessions analyzed (Table 1 and Supplementary Figure 2 ). These data suggest that it is likely that Ping was selected against or lost from most accessions during the hypothesized two or more domestication events from O. rufipogon populations [10] , [14] . Fig. 2 Copy numbers of mPing, Ping , and Pong elements in rice subgroups. a mPing copy numbers in 3000 genomes and the four accessions undergoing mPing bursts (HEG4, EG4, A119, and A123). Colors represent the five major rice subgroups: indica (IND), aus/boro (AUS), aromatic (ARO), temperate japonica (TEJ), tropical japonica (TRJ), and admixed (ADM). b Ping copy numbers in 3000 genomes and the four accessions undergoing mPing bursts. c Neighbor-joining tree of temperate japonica accessions using genome-wide SNPs. d mPing copy number of temperate japonica accessions. e Ping copy number of temperate japonica accessions. Accessions that have the Ping16A_Stow locus are noted with open circles. Source data for Fig. 2a, b, d, e are provided in Supplementary Data 1 Full size image Table 1 Distribution of Ping variants and Ping16A_Stow genotypes in domesticated rice and O. rufipogon Full size table Origin of a Ping variant and its possible significance Analysis of the extensive collection of rice genomes revealed that a SNP distinguishing Ping and mPing ( + 16 G/A), located adjacent to the 15-bp terminal inverted repeat (TIR) (Fig. 3a ), may be implicated in mPing bursts. Pings having these SNPs are distinguished herein as Ping16G (identical shared sequences with mPing ) and Ping16A . First, all 21 O. rufipogon accessions with Ping have only Ping16G , which has the same sequence at + 16G/A as mPing (Table 1 ). Thus, Ping16G is the original Ping and all four mPing subtypes ( mPingA-D , Supplementary Table 2 ) arose prior to domestication by internal deletion. Second, of the 199 domesticated rice accessions with Ping , 31 have Ping16G , whereas 154 have Ping16A (Table 1 ). The presence of the derived Ping16A in both indica and japonica accessions was initially confusing as it suggested the unlikely scenario that this variant arose independently during or after the hypothesized two domestication events that led to these subspecies [10] , [14] . However, closer examination of local sequence ancestry revealed that, where a determination could be made, all of the Ping16A loci in indica and admixed accessions originated by introgression from japonica (Table 1 ). Thus, Ping16A has experienced limited but significant proliferation during or after japonica domestication such that it now accounts for the majority of Ping elements present in domesticated rice accessions (Table 1 ). Fig. 3 Transposition frequency of mPing variants in the yeast assay. a Sequence alignment of mPing and Ping16A terminal sequence (1–40 bp). The SNP between mPing and Ping16A at position 16 ( + 16 G/A SNP) is indicated by the red arrow. b Transposition frequency of mPing variants with mutations at the 5ʹ end in the yeast assay. X axis indicates mPing variants with mutations at 14 positions in the 5ʹ TIR and two positions outside the TIR. For example, mPingG16A represents an mPing variant having a G-to-A mutation at position 16. A variant mPingC4A was not included because the lack of qualified experiments. Y axis shows transposition frequency that was measured as mPing excision events per million cells and normalized to the control mPing . The error bars show standard deviation (s.d.) of 2-9 independent biological replicates. Letters (a and b) above the bars indicate significant differences of transposition frequency between mPing variants and control (adjusted P -value ≤ 0.05). The adjusted P- values are based on a one-way ANOVA ( P- value = 2.37e–15, F- value = 12.34, DF = 16) followed by a Tukey’s honest significant difference (Tukey’s HSD) test. Source data for Fig. 3b are provided as a Source Data file Full size image Reduced mobility of Ping16A in yeast assays The TIRs and adjacent sequences of several DNA transposons have been shown to be functionally significant with mutations of these sequences reducing transposition frequency by decreasing the binding of transposase [23] , [24] . Because the SNP distinguishing Ping16A from Ping16G is adjacent to the 15-bp 5ʹ TIR (Fig. 3a ), we employed a yeast assay to assess transposition rates of 14 mutations within and 2 mutations adjacent to the 5ʹ TIR (Fig. 3b ). In this assay, Pong transposase and an enhanced Ping ORF1 (the putative binding domain) catalyzes transposition of mPing inserted in an ADE2 reporter gene, thereby allowing growth of yeast cells [18] , [25] . The results indicate that both the mutations adjacent to the TIRs (G16A and G17T) and 12 of 14 mutations in the TIR significantly reduced mPing transposition (one-way ANOVA with Tukey’s HSD test, adjusted P -value ≤ 0.05; Fig. 3b ), supporting the hypothesis that this SNP ( + 16 G/A) may have functional significance by reducing Ping16A ’s mobility. Although Pong transposase, which was shown previously to catalyze higher transposition frequency than Ping , was used in this experiment to facilitate the yeast transposition assays, its catalytic mechanism is likely indistinguishable from Ping transposase [25] . Furthermore, the reduced transposition of the G16A mutant ( mPingG16A ) was independently confirmed using Ping transposase (Supplementary Figure 5 ). A Ping locus correlates with higher mPing copy number The four accessions previously shown to be undergoing mPing bursts (HEG4, EG4, A119, A123) have many (7–10) Pings , and all share only a single Ping , Ping16A_Stow [7] . This correlation suggests that acquisition of Ping16A_Stow may have initiated the burst. Ping16A_Stow , located on chromosome 1 (2640500–2640502), is comprised of the Ping16A variant inserted in a 769-bp Stowaway element (Fig. 4a ). Of interest was whether any of the 3000 accessions had Ping16A_Stow and, if so, did they also have more mPings . Fig. 4 Structure of the Ping16A_Stow locus, which is associated with increased mPing copy number. a Structure of the Ping16A_Stow insertion site. The Ping16A element (green arrow) is inserted in the middle of a nonautonomous Stowaway element (red box), which is not in Nipponbare (blue bar). Nucleotides shown within the blue dotted lines are the sequences of the nonautonomous Stowaway element. Target site duplications (TSDs) are indicated by nucleotides underscored. b Comparisons of mPing copy number in 3000 rice accessions with or without Ping16A_Stow in the genome. Gray dots indicate mPing copy number of rice accessions in each category. The error bars show standard deviation (s.d.) of each category. Differences in mPing copy numbers between two categories were tested by a two-tailed Wilcoxon–Mann–Whitney test. Source data for Fig. 4b are provided in Supplementary Data 1 Full size image Among the 3000 accessions, 11 have Ping16A_Stow (188 have only the Stowaway insertion at this locus) (Table 1 ) and these accessions have significantly more mPings (two-tailed Wilcoxon–Mann–Whitney test, P = 2.5e–08; Fig. 4b , Table 2 , and Supplementary Table 3 ), providing additional correlative evidence for the involvement of Ping16A_Stow in mPing bursts. Table 2 Ping copy numbers and genotypes in rice accessions with high copy numbers of mPing Full size table Pong has been stably silenced since domestication Pong encoded proteins catalyze transposition of mPing in yeast and A. thaliana assays [17] , [18] and in rice cell culture [5] . However, because Pong elements are epigenetically silenced in Nipponbare and in accessions undergoing mPing bursts (HEG4, EG4, A119, A123) [7] , there is no evidence to date that Pong has an impact on Ping or mPing copy number or distribution. Data from this study extend previous findings [7] and suggest that Pong was silenced in O. rufipogon and has been stably silenced in domesticated rice. Pong elements are present in the genomes of almost all of the analyzed rice accessions (99.1%, 2972/3000), and Pong copy numbers vary little within or between subgroups (Supplementary Figure 6 ). On average, rice accessions have four Pong elements (Fig. 1d ). All O. rufipogon accessions have Pong elements (Supplementary Figure 2 ), except four (W1849, W1850, W2022, W2024), which appear to contain only Pong deletion derivatives (see Methods). As in domesticated rice, there is minimal Pong copy number variation among the O. rufipogon accessions examined (Supplementary Figure 2 ). Six rice accessions with higher Pong copy numbers (14–25) were analyzed to determine if this resulted from Pong activation. First, because active Pong elements produce proteins that catalyze mPing transposition, we tested if the genomes of these lines contained more mPings . However, all six accessions had the same range of mPing copies as accessions with few Pongs (Supplementary Table 4 ). Second, because host regulatory mechanisms suppress transposition, other potentially active TEs (elements shown previously to transpose when epigenetic regulation is impaired) may have been activated in these accessions along with Pong . However, the six accessions harbored average copy numbers of nine potentially active TEs (Supplementary Table 4 ). Taken together these data suggest that these six accessions have accumulated silenced Pong elements since domestication. Finally, additional evidence for the stability of Pong silencing can be inferred from the observation that none of the 2801 accessions lacking Ping have a higher mPing copy number than accessions with Ping . Results of the evolutionary inventory of the members of the mPing/Ping/Pong TE family in wild and domesticated rice genomes suggest the following scenario for the origin of the mPing burst. All mPing subtypes in domesticated accessions ( mPingA-D ) were generated prior to domestication, probably in O. rufipogon , by internal deletion from Ping16G . Furthermore, Ping16G , but not Ping16A , was detected in 21 of 48 O. rufipogon accessions. The fact that only 31 of the 3000 extant domesticated accessions examined have Ping16G suggests that there has been a massive loss of this element in domesticated rice. In contrast, the Ping16A variant was identified in the majority of the domesticated accessions with Ping (154/199). Its absence in O. rufipogon genomes indicate that it was either very rare in wild populations or that it arose in japonica after domestication. Ping16A has experienced limited but significant proliferation in japonica and has even been introgressed into a small number of indica accessions (Table 1 ). Taken together, these data indicate that Ping16A has become more widely distributed in domesticated accessions, whereas Ping16G is disappearing. Yeast assays testing the functional impact of several mutations in and adjacent to the Ping TIR demonstrate that the + 16G ( Ping16G ) to + 16A ( Ping16A ) polymorphism significantly reduces transposition frequency. Thus, Ping16A encoded proteins (which are identical to Ping16G encoded proteins) are more likely to catalyze the transposition of mPing (with its + 16G) than Ping16A . This situation is reminiscent of other autonomous elements that harbor sequences that reduce transposition frequency [26] , [27] . It has been hypothesized that autonomous TEs enhance their survival by evolving self-regulating mutations that reduce both host impact and epigenetic detection and silencing [27] . The vast majority of accessions with Ping16A have only one Ping (105/154 accessions) and a moderate number of mPing elements (mean = 28). One of these accessions is the reference accession Nipponbare where the inability to detect transposition of Ping or mPing was initially attributed to Ping silencing [28] . In fact, Ping is not silenced in Nipponbare nor in any other accession analyzed to date [7] . Rather it is transcribed and catalyzes (infrequent) transposition of mPing [6] , [7] . We speculate that accessions with a single copy of Ping16A may be experiencing a balance, perhaps under stabilizing selection, between host survival and the maintenance of an active TE family in the genome. The hypothesized balance between Ping16A and mPing elements and the host was perturbed in the subset of temperate japonica accessions experiencing mPing bursts [7] and it was suggested that the shared Ping16A_Stow locus may have been responsible [7] . Based on the evolutionary inventory presented in this study, it follows that Ping16A_Stow was generated in a temperate japonica accession when Ping16A transposed into a Stowaway element on chromosome 1. The Stowaway element (without the Ping insertion) was also present at this locus in O. rufipogon (Table 1 ). It is unlikely that this Stowaway is active as there are only four family members, each with < 96% sequence identity, in the Nipponbare genome. Here we find that Ping16A_Stow is also shared by five of the six accessions with the highest mPing copy numbers among the 3000 accessions analyzed (Table 2 ). The sixth accession, IRIS_313_15904, has a region of introgressed indica or aromatic alleles at this location, which may have replaced the Ping16A_Stow locus in prior generations. The association of Ping16A_Stow with higher mPing copy numbers is consistent with its suggested role in triggering mPing bursts. However, the mechanism by which Ping16A_Stow may initiate the burst is unknown and warrants further investigation. Prior studies indicated that increased Ping transcripts were correlated with more mPing transpositions in accessions undergoing mPing bursts [7] , [28] . Our unpublished data suggest that Ping16A_Stow does not produce more transcripts compared with other Ping elements, suggesting that mechanisms other than an increased transcript level from this locus may be responsible. In conclusion, the results of this study demonstrate that mPing bursts are likely restricted to the past century as none of the thousands of genomes analyzed have as many mPing (hundreds) and Ping (7–10) elements as the four previously characterized accessions. Further, analysis of the 3000 rice genomes and wild progenitors indicates that two variants of the autonomous Ping element, Ping16A and the subsequently evolved Ping16A_Stow locus appear to be critical for mPing hyperactivity. Other studies have shown that domestication can be associated with the loss of epigenetic regulation [29] , which may lead to the activation of TEs. However, our data indicate that Pong element copy number has been stably maintained from the wild ancestor through the generation of the thousands of domesticated accessions, suggesting that epigenetic regulation was unaffected. In contrast, Ping activity has been sustained during domestication, resulting in the spread and amplification of the Ping16A variant and the generation of the Ping16A_Stow locus in rice. Yet, the spread of Ping activity associated with exceptional mPing activity has been very limited in rice, likely due to its high level of self-fertilization. Dataset Illumina DNA sequencing reads of 3000 rice accessions were obtained from NCBI SRA project PRJEB6180. The metadata incorporating name and origin of the 3000 rice accessions was extracted from previously published Tables S1A and S1B [20] . The raw reads of 48 O. rufipogon accessions were obtained from NCBI SRA under project accession numbers listed in Supplementary Data 2 . The metadata associated with the subgroup classification of these 48 O. rufipogon accessions was extracted from prior studies [10] , [30] . The raw reads of Oryza glaberrima , Oryza glumaepatula (also known as Oryza glumipatula ), and Oryza meridionalis were obtained from NCBI SRA projects accession numbers SRR1712585, SRR1712910, and SRR1712972. Population structure and ancestral component analysis The genotyped SNP dataset (release 1.0 3 K RG 4.8 million filtered SNP Dataset) of the 3000 rice genomes was obtained from SNP-Seek Database [31] ( http://snp-seek.irri.org ). A subset of 270,329 SNPs was selected by removing SNPs in approximate linkage equilibrium using plink v1.09 (--indep-pairwise 1000 kb 20 kb 0.8) [32] . Population clustering analysis was performed by ADMIXTURE v1.3.0 [33] (-s 2) with K from 2 to 10. Most rice accessions clustered into five subgroups ( indica : IND, aus / boro : AUS, aromatic ( basmati / sadri ): ARO, temperate japonica : TEJ, and tropical japonica : TRJ) when K is 5. Using the ancestral analysis of ADMIXTURE under the K = 5 model, a rice accession was assigned to one of these five subgroups if it had ≥ 80% of its ancestral component from a given subgroup. Any accessions that had no major ancestral component ( < 80%) were categorized as admixed (ADM) accessions. During the preparation of this study, Wang et al. published an analysis of the same dataset [14] . The subgroup classifications were compared between the two studies and the results are consistent except that Wang et al. identified additional subgroups in indica and japonica . The 4.8 million filtered SNPs were imputed and phased with BEAGLE v5.0 [34] using default parameters (impute = true imp-states = 1600 imp-segment = 6.0 cluster = 0.005). A total of 768 accessions with major ancestral component over 99.99% were used as reference panels for five rice subgroups (344 indica accessions, 111 aus/boro accessions, 31 aromatic accessions, 124 temperate japonica accessions, and 158 tropical japonica accessions). Local ancestry assignment was performed on accessions of interest with RFMix v2.03 [35] using default parameters. Regions of interest were manually inspected in the results of RFMix. Introgression was defined as an allele that is present in one subgroup but has originated from another subgroup. Copy numbers characterization The mPing , Ping , and Pong insertion sites across the 3000 rice genomes were characterized with RelocaTE2 (aligner = BLAT mismatch = 1 len_cut_trim = 10) [19] using raw reads obtained from NCBI SRA. Element-specific sequence differences were identified and used to distinguish Ping and Pong from mPing insertions (Fig. 1a ). Three separate runs of RelocaTE2 were performed using mPing , Ping , and Pong as queries. Paired-end reads where one read of a pair matched the internal sequence of a Ping element (253–5164 bp) and the mate matched to a unique genomic region of the Nipponbare reference genome (MSU7) were used to differentiate Ping insertions. Similarly, paired-end reads where one read matched the internal Pong element sequence (23–5320 bp) and the mate matched to a unique genomic region of MSU7 were used to identify Pong insertions. An equivalent approach was undertaken with mPing sequences but the prior identified Ping and Pong insertion sites were removed from the mPing RelocaTE2 results to generate final mPing insertions. RelocaTE2 analysis was performed in 48 O. rufipogon genomes to identify mPing , Ping , and Pong insertions. However, the short insert size and insufficient read depth of O. rufipogon sequencing libraries prevented distinguishing Ping and Pong insertions from mPing . Copy numbers of mPing , Ping , and Pong elements were estimated from the ratio of the element read depth to the genome-wide average read depth using the script “Rice3k_copy_number_depth_window_mPing/Ping.py”. The genome average sequence coverage for each genome was calculated using qualimap v2.1.2 [36] . The element read depth was calculated using a window-based approach to capture read depth variation across the element. All sequencing reads associated with a given repeat element were extracted from the RelocaTE2 results. The reads were aligned to the element using BWA v0.7.12 [37] with default parameters (mem -k 19 -w 100 -T 30). Alignments with ≤ 2 mismatches were retained for further analysis. The sequence coverage of each position in the element was calculated using mpileup command in SAMtools v0.1.19 [38] (mpileup -d 8000). Positions 1–430 bp of mPing element was divided into 50-bp windows with 40-bp of overlapping sequence between adjacent windows. The read depth of each 50-bp window of mPing was extracted from mpileup results. The copy number of each 50-bp window was defined as the ratio of the depth of each 50-bp window to the genome-wide average read depth. Approximate estimation of mPing copy numbers was from an average copy number of all 50-bp windows. Ping and Pong copy numbers were calculated using positions 260–3260 bp so that unique regions in the targeted element were considered for the assessment. To confirm the statistical differences a one-sample t -test was performed to determine whether the average read depth of 50-bp windows of a given element was equal to genome-wide average read depth. The read depth method was evaluated using simulated datasets. Simulated TE insertions were generated by randomly inserting mPing elements into rice chromosome 3 (OsChr3) and chromosome 4 (OsChr4) using custom scripts. Copy numbers of 1, 10, 100, and 1000 mPing s were simulated to evaluate the performance of the read depth on TE copy numbers. Three replicates were generated for each dataset. Sequencing datasets were simulated with pIRS [39] at varying depths of 1, 2, 3, 4, 5, 10, 20, and 40 to evaluate the performance of the read depth method on sequencing depths. Sequencing reads were aligned to OsChr3 and OsChr4 with SpeedSeq [40] (align -t 24 -R “@RG/tID:id/tSM:sample/tLB:library”), which uses BWA (mem -k 19 -w 100 -T 30) to align reads, Sambamba [41] (-M 20) to sort alignments, and SAMBLASTER [42] (-c 2 -m 20) to mark PCR duplicates. Genome-wide sequencing depths were obtained with qualimap using BAM files generated by SpeedSeq. mPing -related reads were obtained with RelocaTE2 (--size 500 --mismatch 2 --aligner blat) and were aligned to mPing sequence with BWA (mem -k 19 -w 100 -T 30). Alignments with ≤ 2 mismatches were retained for further analysis. The sequence coverage of each position in the element was calculated using mpileup command in SAMtools (mpileup -d 100000). mPing copy numbers were characterized with the script “Rice3k_copy_number_depth_window_mPing.py”. The results indicate that the read depth method can estimate approximate mPing copy numbers with a wide range of sequencing depth (Supplementary Figure 7 ). Even at a low coverage of 2 where RelocaTE2 shows low efficiency to identify TE insertions, the read depth method can accurately estimate mPing copy number when there is only a single element in the genome (Supplementary Figure 7a ). The presence and absence of mPing , Ping , and Pong were also confirmed with manual inspection. Briefly, mPing , Ping , and Pong -associated reads were extracted and aligned to the elements as described above. The sequence coverage of mPing , Ping , and Pong were inspected using heatmap and Integrative Genomics Viewer (IGV) v2.3.0 [43] . Only accessions showing sequence coverage across a given element (generally needs ≥ 70% of elements covered) were defined as accessions having this element. This approach was also used to identify four Aus / boro accessions that have a Ping locus (Chr11: 25822230–25802232) that was not identified with RelocaTE2. Analysis of Ping16A_Stow The pre-aligned BAM files of 3000 rice genomes ( http://s3.amazonaws.com/3kricegenome/Nipponbare/ ”Accession_Name”.realigned.bam) were analyzed to determine if a Stowaway element was present at the Ping16A_Stow locus Chr1: 2640500–2640502. A total of 199 rice genomes with signatures of TE insertions at the Ping16A_Stow locus (reads with only partial “soft clipped” alignments) were analyzed to confirm the Stowaway insertion. A pseudogenome was built of a single Stowaway element and its 2-kb flanking sequences at position Chr1: 2640500–2640502. The sequencing reads from each of the 199 rice genomes were aligned to the pseudogenome using BWA with default parameters (mem -k 19 -w 100 -T 30) followed by analysis of the BAM files to identify junction reads covering both the Stowaway and its flanking sequence. All of these 199 accessions were confirmed to have the Stowaway element at position Chr1: 2640500–2640502. A similar approach that identified the Stowaway insertion was used to identify Ping insertions in the Stowaway element at the Ping16A_Stow locus. A pseudogenome was built using a Ping element and its flanking sequences, which are 1–305 bp of the Stowaway element upstream of Ping and 306–770 bp of the Stowaway element downstream of Ping . The sequencing reads of these 199 rice genomes were aligned to the pseudogenome using BWA with default parameters (mem -k 19 -w 100 -T 30). Analysis of junction reads covering both Ping element and its flanking Stowaway element identified eleven accessions having a Ping insertion in the Stowaway element at the Ping16A_Stow locus (Supplementary Table 3 ). Analysis of + 16 G/A SNP genotype A locus-specific approach was used to analyze the genotype of the + 16 G/A SNP of the Ping element in rice. Ping -containing reads of each locus were extracted from the RelocaTE2 results and the reads were aligned to the Nipponbare Ping element using BWA with default parameters (mem -k 19 -w 100 -T 30). Alignments with ≤ 2 mismatches were analyzed using mpileup command in SAMtools (mpileup –d 8000) to generate a read depth profile, which includes base composition information at each position. The nucleotide counts at the + 16 G/A SNP were obtained from the read depth profile. A Ping with two or more reads supporting G was genotyped as Ping16G , whereas a Ping locus with two or more reads supporting A was genotyped as Ping16A . The genotypes of three Ping loci, including Chr6: 23521641–23526981 (Nipponbare Ping ), Chr1: 264050–2640502 ( Ping16A_Stow ), and Chr11: 25822230–25802232 (a Ping locus in Aus / boro ), were assigned through manual inspection because these loci were either reference Ping (53 accessions with Nipponbare Ping ) or nonreference Ping but have not been identified with RelocaTE2 (11 accessions with Ping16A_Stow and 4 accessions with the Aus / boro Ping locus). For O. rufipogon , all reads aligning to mPing , Ping , and Pong were pooled to analyze the base composition at the + 16 G/A SNP because mPing , Ping , and Pong insertions could not be efficiently sorted. An O. rufipogon genome was categorized as a genome having Ping16G or Ping16A based on whether they had two or more reads supporting G or A. Accessions that have two or more reads supporting both G and A were further analyzed to clarify whether the Ping16A is present in these genomes. For example, accession W1230 had both G (288 reads) and A (23 reads) at the + 16G/A SNP. These A-supporting reads and their mates were extracted from W1230 sequences and aligned to pseudogenomes that have W1230 mPing or Ping inserted in MSU7. All of these A-supporting reads were uniquely aligned to mPing locus Chr3: 25526483–25526485 that contains a 430-bp mPingC element successfully assembled from locus-specific paired-end reads, suggesting these A-supporting reads were from mPing not from Ping . Assembly and classification of mPing sequences A locus-specific assembly was performed to recover full-length mPing sequences from rice sequences. The sequencing reads matching mPing were obtained using RelocaTE2, assembled using velvet v1.2.09 (MAXKMERLENGTH = 31 -ins_length 500 -exp_cov auto -scaffolding yes) [44] . The flanking non- mPing sequences were removed from the assembled sequences. Any mPing candidate loci containing sequence gaps were removed from the analysis. The remaining full-length mPing sequences were compared using BLAST v2.2.26 to build an undirected graph with python package NetworkX ( https://networkx.github.io ). Each node in the graph is an mPing sequence and each edge is a connection, which requires two mPing sequences are properly aligned (number of gaps or mismatches ≤ 4). The mPing sequences in each subgraph represent a subtype of mPing . Representative sequences were extracted from each mPing subtype and aligned with four canonical defined mPing subtypes ( mPingA , mPingB , mPingC , and mPingD ) from the prior study [5] using MUSCLE v3.8.425 [45] with default parameters (-maxiters 16). The multiple sequence alignment in MSA format was converted into VCF format using msa2vcf.jar tool ( https://github.com/lindenb/jvarkit ) to identify polymorphic sites. The assembled mPing sequences were classified into subtypes based on their breakpoints and point mutations compared with the four canonical mPing subtypes. The reads of O. rufipogon accessions were aligned to four canonical defined mPing subtypes ( mPingA , mPingB , mPingC , and mPingD ) using BWA with default parameters (mem -k 19 -w 100 -T 30). Alignments with ≤ 2 mismatches were manually inspected using IGV v2.3.0 to determine if the reads cover breakpoint of each mPing subtype in each accession. An accession with two or more reads covering the breakpoint of an mPing subtype was identified as an accession containing this mPing subtype. Phylogenetic analysis The 270,329 SNPs used for ADMIXTURE analysis were used to genotype HEG4, EG4, A119, and A123 using GATK UnifiedGenotyper v3.4-46 [46] . The phylogenetic tree of rice accessions was built using a neighbor-Joining method implemented in FastTree v2.1.10 (-noml -nome) [47] . The sequencing reads for the 48 O. rufipogon accessions were analyzed to obtain a SNP dataset. Briefly, paired-end reads were aligned to MSU7 using SpeedSeq v 0.1.0 (align -t 24 -R “@RG/tID:id/tSM:sample/tLB:library”). The resulting BAM files were analyzed with GATK UnifiedGenotyper to perform SNP calling. Filtering parameters (QD < 2.0, MQ < 40.0, FS > 60.0, AF < 0.05, HaplotypeScore > 13.0, MQRankSum < –12.5, ReadPosRankSum < –8.0, MQ0 > = 4 && ((MQ0/(1.0×DP)) > 0.1), QUAL < 30.0, DP < 6, DP > 5000, HRun > 5) were used to retain high-quality SNPs using GATK VariantFiltration. Only homozygous SNPs that did not overlap the repetitive sequences were used in the phylogenetic analysis. These high-quality SNPs were extracted and converted into PHYLIP format multiple sequence alignment for phylogenetic analysis with RAXML v8.2.8 [48] under a GTRGAMMA model (-m GTRGAMMA). Bootstrap was performed using 100 iterations (-f a -# 100). O. glaberrima , Oryza glumaepatula , and O. meridionalis were treated as outgroups. Graphical representations of the phylogenetic trees were generated in R using “APE” libraries [49] . Yeast transposition assay mPing was amplified with Phusion High-Fidelity PCR Master Mix (Thermo Fisher Scientific) using the control mPing primers ( mPing F and mPing R) or mutation containing primers (i.e., mPing F and mPing16A R; Supplementary Table 5 ). The primary PCR products were then amplified with ADE2 TSD F and ADE2 TSD R primers (Supplementary Table 5 ) to add ADE2 homologous sequences. Purified PCR products were co-transformed into Saccharomyces cerevisiae strain JIM17 [50] with Hpa I digested pWL89a plasmid using the lithium acetate/polyethylene glycol method [51] . Plasmids were isolated from individual yeast clones using the Zymo Yeast Plasmid Miniprep kit (Zymo Research) and transformed into Escherichia coli for plasmid purification and sequence validation. Sequence verified plasmids were transformed into S. cerevisiae strain CB101 [50] containing previously described pAG413 GAL ORF1 Shuffle1 NLS and pAG415 GAL Pong TPase L384A, L386A plasmids [25] . The transposition rate was measured as described in the prior study [18] . Briefly, 3 ml cultures were grown in CSM-His-Leu-Ura (dextrose) for 24 h at 30 °C, and 100 µl was plated onto 100 mm CSM-His-Leu-Ura-Ade (galactose) plates. The total number of yeast cells was calculated by plating a 10 -4 dilution of the cultures onto YPD plates. The numbers of colonies on the galactose plates were determined after 10 days of incubation at 30 °C. The transposition rate was determined by dividing the galactose colony count by the total number of cells plated. Statistical analysis Sample sizes, statistical tests, and P- values are indicated in figures or figure legends. Linear regression, two-tailed Pearson’s correlation, two-tailed Wilcoxon–Mann–Whitney, one-way ANOVA and Tukey’s HSD test were performed with “lm”, “cor.test”, “wilcox.test”, “aov”, and “TukeyHSD” functions in R. One-sample t -test was performed with ‘ttest_1sample’ function in Python module ‘sci.stats’. Code availability RelocaTE2 and other code used in this study are available at https://github.com/stajichlab/Dynamic_rice_publications or https://doi.org/10.5281/zenodo.1492794 .